Spatial association with PTEX complexes defines regions for effector export intoPlasmodium falciparum-infected erythrocytes Export of proteins into the infected erythrocyte is critical for malaria parasite survival. The majority of effector proteins are thought to export via a proteinaceous translocon, resident in the parasitophorous vacuole membrane surrounding the parasite. Identification of the Plasmodium translocon of exported proteins and its biochemical association with exported proteins suggests it performs this role. Direct evidence for this, however, is lacking. Here using viable purified Plasmodium falciparum merozoites and three-dimensional structured illumination microscopy, we investigate remodelling events immediately following parasite invasion. We show that multiple complexes of the Plasmodium translocon of exported proteins localize together in foci that dynamically change in clustering behaviour. Furthermore, we provide conclusive evidence of spatial association between exported proteins and exported protein 2, a core component of the Plasmodium translocon of exported proteins, during native conditions and upon generation of translocation intermediates. These data provide the most direct cellular evidence to date that protein export occurs at regions of the parasitophorous vacuole membrane housing the Plasmodium translocon of exported proteins complex. Malaria disease places a major global burden on human health. It is caused by protozoan parasites from the genus Plasmodium , with P. falciparum causing the most severe form in humans. All associated pathologies derive from the blood stage lifecycle, when the parasite develops and divides within circulating erythrocytes [1] . Erythrocyte infection is established by blood-stage merozoites, the smallest parasite lifecycle stage. During invasion the merozoite becomes surrounded by a membranous compartment, the parasitophorous vacuole (PV) [2] . The parasite then initiates a remarkable remodelling process, converting the terminally differentiated erythrocyte that lacks basic machinery for protein trafficking, into one in which it can obtain all nutrients necessary for growth, development and replication (reviewed in Marti et al . [3] ). Modulation of virulence-associated properties, including erythrocyte rigidity, cytoadherence and presentation of virulence-associated antigens on the erythrocyte surface occur at this time [4] , [5] , [6] . Remodelling requires export of hundreds of parasite-derived proteins across the PV membrane (PVM) into the host cell [7] , [8] , [9] . This requires establishment of protein trafficking and sorting machinery that facilitates the movement of proteins onto and under the erythrocyte membrane [10] , [11] . A common feature of many exported proteins is the presence of a hydrophobic N-terminal signal sequence, followed by a pentameric motif (RxLxE/Q/D) called the Plasmodium export element (PEXEL) [7] /vacuolar transport sequence (VTS) [8] . An endoplasmic reticulum resident protease, plasmepsin V, cleaves this motif, targeting the protein for export [12] , [13] and recently binding to phosphitidylinositol-3-phosphate moieties has been implicated [14] . Export is ATP-dependent and requires protein unfolding, suggesting that transport occurs through a proteinaceous translocon at the PVM [7] , [15] . A PVM-associated complex has been identified with the expected properties of a translocon machine [16] . This putative P. falciparum translocon of exported proteins (PTEX) consists of at least five proteins: exported protein 2 (EXP2), PTEX 150 (PTEX-150), heat-shock protein 101 (HSP101), thioredoxin 2 (TRX2) and PTEX 88 (PTEX-88), which exist in a stable macromolecular complex of >1,230 kDa [17] . EXP2, a membrane-associated protein with a fold similarity to the pore forming toxin Escherichia coli haemolysin E [16] , associates in homo-oligomeric species comprising at least eight separate subunits and interacts more strongly with the PVM than the other known PTEX components [17] . These characteristics are consistent with EXP2 being the pore through which exported proteins pass [16] . However, despite considerable circumstantial evidence there remains no direct evidence for the role of PTEX. Protein translocators have been studied in many systems, particularly eukaryotic organellar import machinery and the bacterial SecYEG export complex [18] , [19] . Characterization of these systems has relied on in vitro biochemical assays and creation of transport mutants that prevent translocation, for example fusion to a dihydrofolate reductase (DHFR) tag. DHFR is prevented from unfolding, and therefore completion of transit, in the presence of antifolate compounds [20] . The intracellular nature of P. falciparum has made the former approach difficult. Fusion of exported malaria proteins to a DHFR domain, however, has demonstrated the importance of protein unfolding for transit [15] . Early imaging studies using the same strategy with transition mutants blocked during mitochondrial and chloroplast import revealed non-uniform patches of translocators in these organelles [21] , [22] , [23] . More recently, high-resolution imaging of the translocase of outer membrane (TOM) complex in mitochondria showed clusters within the mitochondrial membrane and demonstrated dynamics in their association [24] . Here we use three-dimensional structured illumination microscopy (3D-SIM) and purified viable P. falciparum merozoites to localize protein export following erythrocyte invasion. We show core PTEX components are present at the PVM within minutes of invasion, where they are deposited as large, dynamic macromolecular clusters. We present evidence of a clear spatial association between PTEX and exported proteins, both during native export conditions and under translocation inhibition using DHFR-stabilised mutants. This identifies discrete regions at the PVM associated with export and provides prima facie evidence that PTEX is a critical mediator of this essential function. P. falciparum morphology changes post erythrocyte invasion To investigate molecular and morphological events after parasite invasion of erythrocytes we used viable purified P. falciparum merozoites [25] to obtain synchronized ring stage parasites for imaging. Widefield deconvolution microscopy of parasites fixed <12 min after initiation of invasion by indirect immunofluorescence assay (IFA) demonstrated extensive morphological changes had occurred at this stage in the lifecycle ( Fig. 1a ). Co-labelling using markers of the merozoite plasma membrane, merozoite surface protein 1 (MSP1) [26] , and the PV, rhoptry-associated protein 1 (RAP1) [27] , identified two distinct changes: amoeboid-like forms of the intracellular parasite with pseudopodia-like extensions involving both vacuole and plasma membranes, and whorl-like extensions involving only the PVM ( Fig. 1a ). These findings add molecular detail to cellular structures previously observed by electron microscopy in Plasmodium knowlesi and Plasmodium chabaudi [2] , [28] , [29] and by live microscopy in P. falciparum [30] . 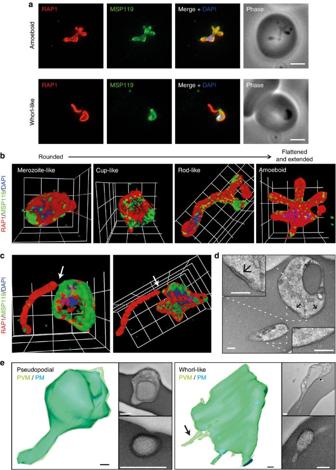Figure 1:P. falciparummerozoite morphology changes post erythrocyte invasion. Parasites were fixed <12 min following merozoite invasion and labelled by IFA using standard markers for the PV (RAP1, red), parasite plasma membrane (MSP1-19, green) and nucleus (4′,6–diamidino-2-phenylindole (DAPI), blue). (a) Widefield deconvolution microscopy identified various morphological changes that had occurred within this period, including pseudopodia-like extensions (top) and whorl-like extensions (bottom). Scale bar, 2.5 μm. 3D-SIM imaging of similarly prepared and labelled parasites confirmed (b) pseudopodia-like and (c) whorl-like morphology changes, showing transitional stages from rounded merozoite-like to more flattened and extended amoeboid forms. Grid=0.5 μm. Gamma settings were altered on images for display purposes only. (d) Transmission electron microscopy (TEM) analysis of parasites <10 min post erythrocyte invasion identified IMC remnants present in cup-like (upper parasite and inset, arrows) and absent in more flattened parasites (lower parasite and inset). Representative section of a doubly infected erythrocyte is shown. Scale bar, 200 nm. (e) 3D modelling of serial sections by TEM confirmed pseudopodia-like (left) and whorl-like PVM (right) extensions. Light green=PVM, darker region=PM. Scale bar, 200 nm. Figure 1: P. falciparum merozoite morphology changes post erythrocyte invasion. Parasites were fixed <12 min following merozoite invasion and labelled by IFA using standard markers for the PV (RAP1, red), parasite plasma membrane (MSP1-19, green) and nucleus (4′,6–diamidino-2-phenylindole (DAPI), blue). ( a ) Widefield deconvolution microscopy identified various morphological changes that had occurred within this period, including pseudopodia-like extensions (top) and whorl-like extensions (bottom). Scale bar, 2.5 μm. 3D-SIM imaging of similarly prepared and labelled parasites confirmed ( b ) pseudopodia-like and ( c ) whorl-like morphology changes, showing transitional stages from rounded merozoite-like to more flattened and extended amoeboid forms. Grid=0.5 μm. Gamma settings were altered on images for display purposes only. ( d ) Transmission electron microscopy (TEM) analysis of parasites <10 min post erythrocyte invasion identified IMC remnants present in cup-like (upper parasite and inset, arrows) and absent in more flattened parasites (lower parasite and inset). Representative section of a doubly infected erythrocyte is shown. Scale bar, 200 nm. ( e ) 3D modelling of serial sections by TEM confirmed pseudopodia-like (left) and whorl-like PVM (right) extensions. Light green=PVM, darker region=PM. Scale bar, 200 nm. Full size image For higher resolution investigation, various super-resolution fluorescence microscopy approaches were explored. Attempts to use continuous-wave stimulated emission depletion microscopy were unsuccessful due to sample damage. The three-dimensional and intracellular nature of the parasite would limit the effectiveness of localization-based techniques. As such, we used 3D-SIM for further analyses. Using 3D-SIM, various ring-stage morphologies were observed <12 min post invasion labelled by anti-RAP1 and anti-MSP1 antibodies. These included rounded merozoite-like, cup-like and more extended and/or flattened discoidal, rod-like and amoeboid appliqué forms ( Fig. 1b ) [2] . Parasites at each stage were observed with whorl-like extensions ( Fig. 1c ). Transmission electron microscopy of serial sections confirmed the plasticity of ring forms from cup-like to more flattened architectures and both parasite plasma membrane-dependent and independent extensions into the infected cell ( Fig. 1d ). The presence of the inner membrane complex in cup-like parasites ( Fig. 1d , upper parasite and inset, arrow) but its absence in more flattened forms ( Fig. 1d , lower parasite and inset) suggested this might be an intermediate between the invading merozoite and later morphologies. PTEX complex components localize to the parasite periphery PEXEL-dependent protein export begins within 10 min of invasion [31] , suggesting the translocon responsible for export must be functional within this timeframe. Therefore, the spatiotemporal localizations of key members of the PTEX complex [16] , putatively responsible for protein export, were followed after erythrocyte invasion. Before and during invasion, PTEX members localize to dense granules [17] . Widefield deconvolution microscopy analysis of <12 min old parasites showed EXP2 fluorescence concentrated in puncta around the periphery of the parasite, marked using RAP1 ( Fig. 2a ). EXP2 staining often coincided with both the tips of pseudopodia-like extensions and the connection point between whorl-like extensions and the parasite’s main body—areas consistently devoid of RAP1 staining ( Fig. 2a arrows). Attempts to localize PTEX-150 using either antisera or a haemagglutinin (HA) tagged copy of the protein were unsuccessful using this method. Therefore, the integrity of the PTEX complex was investigated following invasion using parasites expressing HSP101HA [16] . We performed a time course of fixation to yield parasites <10 min post invasion, when low numbers of parasites have begun export, <20 min and <45 min post invasion, when essentially all parasites show signs of export, and 15–16 h post invasion, as a late ring-stage control. Widefield deconvolution microscopy and 3D-SIM analysis of HSP101HA parasites consistently showed coincidental localization between HSP101HA and EXP2 in puncta at the parasite periphery but, in many instances, also labelled more broadly throughout the parasite in either peri nuclear or parasite peripheral locations ( Fig. 2b ). The proportion of signal localized with EXP2 appeared to vary between parasites. To quantify these differences across the lifecycle we used an automated image analysis approach to measure the percentage of HSP101HA signal, as calculated by summed pixel intensities, overlapping with EXP2 (% colocalization) in 3D-SIM data sets ( Fig. 2d ; Table 1 ). This statistic was robust between images, as demonstrated by consistent values arising from multiple independent analyses of the same parasite ( Supplementary Fig. S1 ). At all time points considerable HSP101HA localized with EXP2 ( Table 1 ). Although some pairs of samples showed statistically significant differences (<10 min versus <20 min, P <0.001 and <20 min versus 15–16 h, P <0.01 using Kruskal–Wallis test with Dunn's post test), the magnitudes of such differences were slight and fell within the margins of variation. Therefore, taking both observed and statistical analyses into account, we concluded that HSP101 localization with EXP2 is established within 10 min of invasion and maintained throughout the ring-stage lifecycle. This is consistent with an intact PTEX having a role in export immediately after invasion. 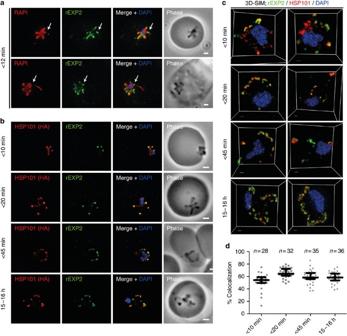Figure 2: PTEX components localize to the parasite periphery immediately following invasion. (a) Widefield deconvolution imaging of parasites fixed <12 min following erythrocyte invasion and labelled by IFA for EXP2 (green), the PV (RAP1, red) and the nucleus (4′,6–diamidino-2-phenylindole (DAPI), blue) showed EXP2 localized in puncta at the parasite periphery at this time point (scale bar, 1 μm). HSP101HA parasites were fixed <10 min, <20 min, <45 min and 15–16 h following erythrocyte invasion and labelled by IFA for EXP2 (green), HSP101HA (HA, red) and the nucleus (DAPI, blue). (b) Widefield deconvolution microscopy (scale bar, 1 μm) (aandb) and (c) 3D-SIM imaging (scale bar, 300 nm) both showed the presence of substantial regions of coincident fluorescence between EXP2 and HSP101HA (scale bar, 0.3 μm). (d) The percentage signal overlap (% colocalization), measured as the sum of pixel intensities, was quantified between HSP101HA with EXP2-labelled regions in 3D-SIM data sets across the time course period (<10 min,n=28; <20 min,n=32; <45 min,n=35; 15–16 h,n=36). Graph shows median with interquartile range. Statistics can be found inTable 1. Figure 2: PTEX components localize to the parasite periphery immediately following invasion. ( a ) Widefield deconvolution imaging of parasites fixed <12 min following erythrocyte invasion and labelled by IFA for EXP2 (green), the PV (RAP1, red) and the nucleus (4′,6–diamidino-2-phenylindole (DAPI), blue) showed EXP2 localized in puncta at the parasite periphery at this time point (scale bar, 1 μm). HSP101HA parasites were fixed <10 min, <20 min, <45 min and 15–16 h following erythrocyte invasion and labelled by IFA for EXP2 (green), HSP101HA (HA, red) and the nucleus (DAPI, blue). ( b ) Widefield deconvolution microscopy (scale bar, 1 μm) ( a and b ) and ( c ) 3D-SIM imaging (scale bar, 300 nm) both showed the presence of substantial regions of coincident fluorescence between EXP2 and HSP101HA (scale bar, 0.3 μm). ( d ) The percentage signal overlap (% colocalization), measured as the sum of pixel intensities, was quantified between HSP101HA with EXP2-labelled regions in 3D-SIM data sets across the time course period (<10 min, n =28; <20 min, n =32; <45 min, n =35; 15–16 h, n =36). Graph shows median with interquartile range. Statistics can be found in Table 1 . Full size image Table 1 ‘Colocalization’ analysis of HSP101 versus EXP2 3D-SIM time course data sets. Full size table EXP2 localization dynamics throughout the ring stage To investigate the nature and dynamics of EXP2 localization in the ring-stage, 3D-SIM imaging was undertaken on parasites fixed <12 min, 60–90 min, 11–12 h and 18-19 h post invasion using antibodies against EXP2 and RAP1. The results indicated that variation in labelling size and distribution occurs both between samples and across the lifecycle ( Fig. 3a ). In earlier time points, multiple foci of fluorescence were apparent, clustered within larger regions of labelling ( Fig. 3b , zoom and arrows) and commonly showing a recurring structure ( Fig. 3c ); however, these clusters were rarely seen in later time points ( Fig. 3a , 11–12 h and 18–19 h time points). To quantify the observed differences across the lifecycle, areas of EXP2 fluorescence were analysed by automated image analysis, using average volume of labelling as an indicator of size. Region-growing algorithms are regularly used to segment adjacent foci. Following region-growing analysis in 3D, which appropriately reflected observed segmentation ( Supplementary Fig. S2 ), the average size of these ‘Segmented’ foci remained relatively constant across time points ( Fig. 3d , green bars; Supplementary Table S1 ), with an overall average size of labelled foci estimated as 0.008±0.002 s.d. μm 3 (parasites n =105). Although acknowledging the limitations in accuracy for this estimate, including the involvement of primary and secondary antibodies (adding ~17.5 nm in each direction), the rejection of subresolution labelled regions during foci identification, potential variations introduced by specific segmentation parameters and microscope resolution limits, this value predicts a region diameter in the order of 200 nm. Even large errors in this measurement would suggest that each focus must contain multiple PTEX complexes. Re-analysis of the same data without use of the segmenting algorithm was next used to investigate the size of the larger ‘Pre-segmentation’ clusters of EXP2 foci. These showed a clear reduction in cluster size occurring with progression through the lifecycle ( Fig. 3d , blue bars; Supplementary Table S1 ). Importantly, both analyses gave similar results in later time points (as visually apparent in Fig. 3a ), with the small disparity attributed to the differences in thresholding protocols used. Taken together, these results demonstrate that individual foci of EXP2 contain multiple PTEX complexes and show dynamics in their clustering, originally deposited in large clusters that progressively spread around the parasite into discrete puncta during the first ~12 h of the asexual lifecycle. 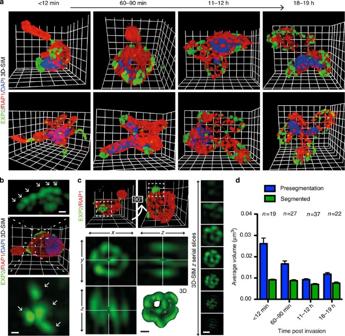Figure 3: EXP2 exhibits clustering dynamics across the ring-stage lifecycle. A time course of parasites fixed <12 min, 60–90 min, 11–12 h and 18–19 h after invasion was labelled by IFA for EXP2 (green), the PV (RAP1, red) and the nucleus (4′,6–diamidino-2-phenylindole (DAPI), blue). (a) 3D-SIM imaging confirmed that EXP2 localized as puncta to the parasite periphery throughout this period. Grid=0.5 μm. Gamma settings were altered on images for display purposes only. (b) EXP2-labelled regions (zooms) from the earlier two time points showed apparent clustering of bright foci (arrows). A representative example is shown. Scale bar, 0.15 μm. (c) In these earlier time points a recurring structural motif was also regularly identified in clusters (upper left). A representative example is presented, with the magnified cluster as orthogonal projection and 3D rendering (lower left) and serial slices (right) shown. Scale bar, 0.15 μm. (d) EXP2-labelled volumes (μm3) were calculated in 3D-SIM data sets (12 min,n=19; 60–90 min,n=27; 11–12 h,n=37; and 18–19 h,n=22) before (‘presegmentation’, blue bars) and after (‘segmented’, green bars) treatment with a region growing algorithm to isolate the previously observed foci within larger regions of fluorescence. Graph shows mean±s.e.m. Statistics can be found inSupplementary Table S1. Figure 3: EXP2 exhibits clustering dynamics across the ring-stage lifecycle. A time course of parasites fixed <12 min, 60–90 min, 11–12 h and 18–19 h after invasion was labelled by IFA for EXP2 (green), the PV (RAP1, red) and the nucleus (4′,6–diamidino-2-phenylindole (DAPI), blue). ( a ) 3D-SIM imaging confirmed that EXP2 localized as puncta to the parasite periphery throughout this period. Grid=0.5 μm. Gamma settings were altered on images for display purposes only. ( b ) EXP2-labelled regions (zooms) from the earlier two time points showed apparent clustering of bright foci (arrows). A representative example is shown. Scale bar, 0.15 μm. ( c ) In these earlier time points a recurring structural motif was also regularly identified in clusters (upper left). A representative example is presented, with the magnified cluster as orthogonal projection and 3D rendering (lower left) and serial slices (right) shown. Scale bar, 0.15 μm. ( d ) EXP2-labelled volumes (μm 3 ) were calculated in 3D-SIM data sets (12 min, n =19; 60–90 min, n =27; 11–12 h, n =37; and 18–19 h, n =22) before (‘presegmentation’, blue bars) and after (‘segmented’, green bars) treatment with a region growing algorithm to isolate the previously observed foci within larger regions of fluorescence. Graph shows mean±s.e.m. Statistics can be found in Supplementary Table S1 . Full size image EXP1 localization in the PVM It is known that various PV proteins, including components of PTEX, reside in detergent-resistant membranes (DRMs) within the parasite [16] , [32] , [33] . We therefore reasoned that proteins might localize together with those from similar DRM fractions even without measurable biochemical interaction. Indeed, when EXP2 localization was compared with that of a DRM-enriched protein, the exported protein 1 (EXP1), clear co-incidence of fluorescence was seen using widefield deconvolution microscopy of parasites fixed <15 min, 60–90 min and 20-21 h post invasion, although EXP1 appeared to become more widely distributed around the PVM in the latter sample ( Fig. 4a ). 3D-SIM imaging of parasites 60–90 min post invasion confirmed their coincidence at this time ( Fig. 4b ) with EXP1 to EXP2 overlap (67.0±1.8% s.e.m. ; n =17) showing similar levels to those seen for HSP101HA <20 min post invasion (65.3±1.4% s.e.m. ; n =32) ( Fig. 4c ; Table 2 ). Comparatively, RAP1, another DRM protein enriched in sucrose fractions [16] and DRM complexes [16] , [32] , [33] both with and without EXP2, showed significantly less overlap at a similar time (14.2±2.0% s.e.m., n =25; P <0.001 by Kruskal–Wallis with Dunn's post test) ( Fig. 4c ; Table 2 ). Indeed, as noted above, RAP1 frequently appeared to be excluded from EXP2-labelled PVM regions. Together these analyses strongly suggest that EXP1 and EXP2 co-exist within distinct regions of the PVM, but that simple DRM-enrichment status does not fully explain this localization. 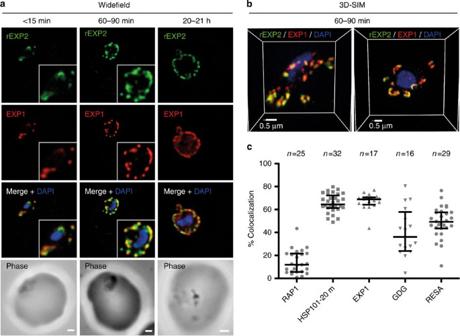Figure 4: EXP1 localizes to PVM domains with PTEX. Parasites were fixed at <15 min, 60–90 min and 20–21 h after invasion and labelled by IFA for EXP1 (red), EXP2 (green) and the nucleus (4′,6–diamidino-2-phenylindole (DAPI), blue). (a) Imaging of all samples by widefield deconvolution microscopy (scale bar, 1 μm), (b) and the 60–90 min sample by 3D-SIM (scale bar, 0.5 μm), suggested strong similarity between EXP1 and EXP2 localizations at the parasite periphery. (c) Using the 3D-SIM data set the percentage overlap (% colocalization), as calculated by the sum of pixel intensities, of EXP1 with EXP2 was calculated (n=17). EXP1 values were comparable with the positive control, HSP101HA <20 min (Fig. 2;n=32) and were substantially higher than the negative control, RAP1 60–90 min (Fig. 3;n=25). Also shown are data measuring percentage of GBP-DHFR-GFP (GDG) (Fig. 5;n=16) and RESA (Fig. 6;n=29) signal overlap with EXP2. Graph shows median and interquartile ranges. Statistics can be found inTable 2. Figure 4: EXP1 localizes to PVM domains with PTEX. Parasites were fixed at <15 min, 60–90 min and 20–21 h after invasion and labelled by IFA for EXP1 (red), EXP2 (green) and the nucleus (4′,6–diamidino-2-phenylindole (DAPI), blue). ( a ) Imaging of all samples by widefield deconvolution microscopy (scale bar, 1 μm), ( b ) and the 60–90 min sample by 3D-SIM (scale bar, 0.5 μm), suggested strong similarity between EXP1 and EXP2 localizations at the parasite periphery. ( c ) Using the 3D-SIM data set the percentage overlap (% colocalization), as calculated by the sum of pixel intensities, of EXP1 with EXP2 was calculated ( n =17). EXP1 values were comparable with the positive control, HSP101HA <20 min ( Fig. 2 ; n =32) and were substantially higher than the negative control, RAP1 60–90 min ( Fig. 3 ; n =25). Also shown are data measuring percentage of GBP-DHFR-GFP (GDG) ( Fig. 5 ; n =16) and RESA ( Fig. 6 ; n =29) signal overlap with EXP2. Graph shows median and interquartile ranges. Statistics can be found in Table 2 . Full size image Table 2 Colocalization’ analysis with EXP2 3D-SIM data sets. Full size table Exported proteins that cannot unfold accumulate with PTEX In the presence of antifolate drugs, such as methotrexate and WR99210 (WR), murine DHFR is unable to unfold [15] , [20] . In this manner, creation of DHFR-fused proteins demonstrated that protein unfolding is essential for malaria parasite protein export [15] . To investigate whether proteins associate with PTEX during export we utilized transgenic P. falciparum parasites expressing a glycophorin binding protein 130 (GBP130) PEXEL-containing leader sequence fused to mDHFR and green fluorescent protein (GBP130-DHFR-GFP) [15] ( Fig. 5a ). WR inhibits export of DHFR-fused proteins in a dose-dependent manner [15] . In our hands, GBP130-DHFR-GFP underwent successful export in the absence of drug but remained within the parasite when grown in the presence of 5 nM WR ( Fig. 5b ), a concentration of drug that did not disrupt the export of native proteins ( Supplementary Fig. S3 ). 3D-SIM analysis of parasites grown without WR and fixed at various stages of GBP130-DHFR-GFP export showed small areas of anti-GFP labelling localized nearby EXP2, but interpretation of the relevance of these was difficult ( Fig. 5c , arrows). We reasoned that, while ultimately export-inhibited protein localized around the entire parasite periphery ( Fig. 5b ) [15] , arrest of trafficking during early stages of GBP130-DHFR-GFP export might allow easily detectable concentrations to form at regions through which export occurs. Indeed, widefield deconvolution microscopy analysis of parasites grown with WR and fixed at 18–19 and 20–21 h post invasion showed regions of clear coincidence between GFP and EXP2 signals ( Fig. 5d ). 3D-SIM investigations of similarly labelled 18–19 h parasites, resolved anti-GFP fluorescence to areas adjacent to regions of EXP2 ( Fig. 5e ; Supplementary Movie S1 ). In the majority, these seemed to localize to the intra-parasitic side of EXP2-labelled domains. Colocalization values for GBP130-DHFR-GFP with EXP2 (40.0±5.2% s.e.m. ; n =16) were low in comparison with those for HSP101HA ( Fig. 4c , Table 2 ); however, broad variance in GBP130-DHFR-GFP results, most likely due to variation in precise fusion protein expression and export stage, prevented statistical analysis. Nevertheless, these observations strongly suggest that blockage of protein unfolding causes accumulation of proteins for export in domains associated with clusters of the PTEX complex. These data are consistent with PTEX acting as a translocon for protein export. 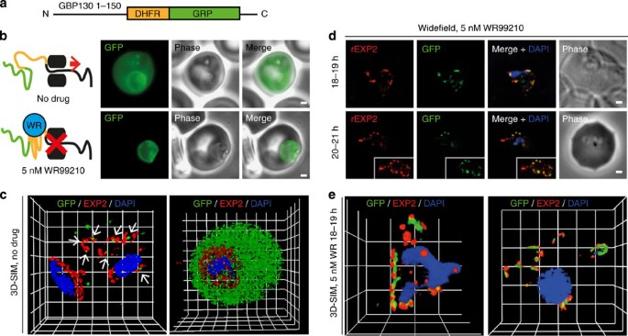Figure 5: Prevention of GBP130-DHFR-GFP protein unfolding causes association with EXP2. (a) The GBP130-DHFR-GFP construct involves a 150 amino-acid leader sequence from the PEXEL containing protein GBP130, fused to mDHFR and GFP. (b) Imaging of live parasites by widefield microscopy showed that the GBP130-DHFR-GFP (GDG, green) reporter was exported in the absence of any drug (top) but was prevented from export when grown in the presence of 5 nM WR99210 (WR) drug (bottom). Scale bar, 1 μm. (c) 3D-SIM imaging of parasites grown in the absence of WR, fixed and labelled by IFA for GBP130-DHFR-GFP (GFP, green), EXP2 (red) and the nucleus (4′,6–diamidino-2-phenylindole (DAPI), blue) demonstrated that analysis of export under native conditions would be difficult using this system. Grid=0.5 μm. Gamma settings were altered on images for display purposes only. Parasites labelled similarly but grown in the presence of 5 nM WR (d) for 18–19 h or 20–21 h and imaged by widefield deconvolution microscopy (scale bar, 1 μm) or (e) for 18–19 h and imaged by 3D-SIM (Grid=0.5 μm; Gamma settings were altered on images for display purposes only) both showed accumulation of translocation intermediates adjacent to areas of EXP2 signal. SeeSupplementary Movie S1for a 3D rotation of the right hand parasite frome. Figure 5: Prevention of GBP130-DHFR-GFP protein unfolding causes association with EXP2. ( a ) The GBP130-DHFR-GFP construct involves a 150 amino-acid leader sequence from the PEXEL containing protein GBP130, fused to mDHFR and GFP. ( b ) Imaging of live parasites by widefield microscopy showed that the GBP130-DHFR-GFP (GDG, green) reporter was exported in the absence of any drug (top) but was prevented from export when grown in the presence of 5 nM WR99210 (WR) drug (bottom). Scale bar, 1 μm. ( c ) 3D-SIM imaging of parasites grown in the absence of WR, fixed and labelled by IFA for GBP130-DHFR-GFP (GFP, green), EXP2 (red) and the nucleus (4′,6–diamidino-2-phenylindole (DAPI), blue) demonstrated that analysis of export under native conditions would be difficult using this system. Grid=0.5 μm. Gamma settings were altered on images for display purposes only. Parasites labelled similarly but grown in the presence of 5 nM WR ( d ) for 18–19 h or 20–21 h and imaged by widefield deconvolution microscopy (scale bar, 1 μm) or ( e ) for 18–19 h and imaged by 3D-SIM (Grid=0.5 μm; Gamma settings were altered on images for display purposes only) both showed accumulation of translocation intermediates adjacent to areas of EXP2 signal. See Supplementary Movie S1 for a 3D rotation of the right hand parasite from e . Full size image Exported proteins associate with EXP2 To extend our observations of parasites fixed under native conditions, we performed widefield deconvolution microscopy, co-labelling EXP2 with antibodies to two key exported virulence proteins, PfEMP3 and PfEMP1. Although both proteins contain PEXEL or PEXEL-like motifs, PfEMP3 traffics in a PEXEL-dependent manner, and PfEMP1 most likely a PEXEL-independent manner. Numerous regions of PfEMP3 fluorescence were co-incident with EXP2-labelled puncta ( Fig. 6a , arrows); however, co-incidence of PfEMP1 and EXP2 labelling was rare at both 11–12 and 18–19 h post invasion ( Fig. 6b , arrows). Although difficult to interpret due to intra-parasitic and non-associated regions of PfEMP3 and PfEMP1 labelling, the result was consistent with PfEMP3 undergoing export through PTEX-marked PVM domains and PfEMP1 trafficking in a PTEX-independent fashion. 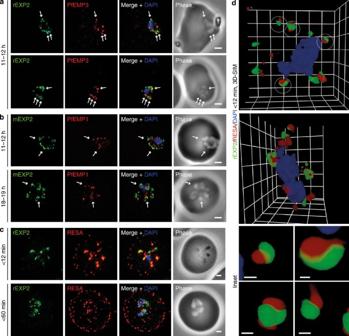Figure 6: Protein accumulates at sites marked by PTEX during native PEXEL-dependent protein export. Widefield deconvolution microscopy of parasites fixed and labelled by IFA for EXP2 (green), the nucleus (4′,6–diamidino-2-phenylindole (DAPI), blue) and (a) PfEMP3 (red), a protein exported by PEXEL-dependent processes, or (b) PfEMP1, a protein likely to undergo PEXEL-independent export, showed some areas of possible association of both exported proteins and EXP2; however, results were inconclusive. Parasite ages are as shown. Scale bars, 1 μm. Parasites were labelled by IFA for EXP2 (green), RESA (red) and the nucleus (DAPI, blue) having been (c) fixed <12 min or 60–90 min after invasion and imaged by widefield deconvolution microscopy (scale bar, 1 μm) or (d) fixed <12 min after invasion and imaged by 3D-SIM (Grid=0.5 μm). Insets show individual PVM domains (scale bar, 0.1 μm) and gamma settings were altered for display purposes only. See alsoSupplementary Movie S2for a 3D rotation of the upper parasite. These results showed that RESA export is detectable in a small proportion of parasite in <12 min assays and in essentially all parasites at 60–90 min. Considerable association, although not direct overlap, was observed between RESA and EXP2 signals at the parasite periphery, particularly in the earlier time point. Figure 6: Protein accumulates at sites marked by PTEX during native PEXEL-dependent protein export. Widefield deconvolution microscopy of parasites fixed and labelled by IFA for EXP2 (green), the nucleus (4′,6–diamidino-2-phenylindole (DAPI), blue) and ( a ) PfEMP3 (red), a protein exported by PEXEL-dependent processes, or ( b ) PfEMP1, a protein likely to undergo PEXEL-independent export, showed some areas of possible association of both exported proteins and EXP2; however, results were inconclusive. Parasite ages are as shown. Scale bars, 1 μm. Parasites were labelled by IFA for EXP2 (green), RESA (red) and the nucleus (DAPI, blue) having been ( c ) fixed <12 min or 60–90 min after invasion and imaged by widefield deconvolution microscopy (scale bar, 1 μm) or ( d ) fixed <12 min after invasion and imaged by 3D-SIM (Grid=0.5 μm). Insets show individual PVM domains (scale bar, 0.1 μm) and gamma settings were altered for display purposes only. See also Supplementary Movie S2 for a 3D rotation of the upper parasite. These results showed that RESA export is detectable in a small proportion of parasite in <12 min assays and in essentially all parasites at 60–90 min. Considerable association, although not direct overlap, was observed between RESA and EXP2 signals at the parasite periphery, particularly in the earlier time point. Full size image To add further clarity towards the visualization of export, we investigated trafficking of the ring-infected erythrocyte surface antigen (RESA). This PEXEL-dependent exported protein is present in dense granules during invasion and exports immediately following invasion. We reasoned that a naturally occurring bottleneck might occur during establishment of the translocon machinery at the PVM, increasing chances of detecting RESA at the location of export. Widefield deconvolution microscopy analysis of parasites <12 min and <60 min post invasion, in agreement with our previous observations [31] , demonstrated detectable RESA export occurring in a small number of<12 min old parasites, and in parasites fixed at later time points ( Fig. 6c ). In <12 min old parasites RESA localized predominantly at the parasite periphery, clearly co-incident with EXP2 ( Fig. 6c , upper panels). At both time points all exported RESA labelling appeared punctate rather than diffuse. Reminiscent of the translocation intermediate analysis, 3D-SIM analysis showed RESA fluorescence commonly localized to regions either immediately to the intra- and/or extra-parasitic side of EXP2 ( Fig. 6d ; Supplementary Movie S2 ). Overlap with EXP2 (49.0±2.5% s.e.m. ; n =29) ( Fig. 4c ; Table 2 ) was significantly higher than RAP1 and lower than HSP101 ( P <0.001 and P <0.01 respectively using Kruskal–Wallis with Dunn's post test). In several instances RESA labelling straddled EXP2 labelling across the PVM or associated within larger clusters of EXP2 ( Fig. 6d , lower panel insets). Taken together with results using the GBP130-DHFR-GFP fusion protein these data strongly suggest that PEXEL-containing proteins traffic through distinct regions of the PVM enriched for PTEX. Identification of PTEX in P. falciparum has suggested it functions as a translocon for effector protein export into the parasite-infected erythrocyte. Although there is considerable circumstantial evidence for an export role for PTEX, as yet there is no direct data [16] . We have used super-resolution imaging and the generation of translocation intermediates to investigate the PTEX complex and its association with effector protein export. This has shown that protein export from the intracellular P. falciparum parasite to the infected erythrocyte occurs through distinct domains in the PV and PVM that involve core PTEX members ( Fig. 7 ). This is the first direct cellular evidence that the PTEX complex functions in P. falciparum protein export. 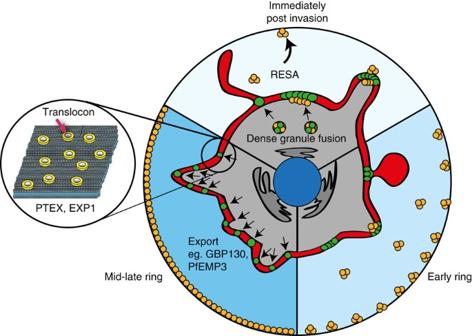Figure 7: Model of export from the ring-stage malaria parasite. Immediately following invasion, dense granule fusion causes local membrane extension and deposits export-associated regions as clusters of foci at the parasite periphery. Each focus contains multiple PTEX complexes as well as non-biochemically associated proteins, such as EXP1. Labelled regions tend to localize at the connexion point to PVM whorl-like extensions and at the tips of pseudopodia-like plasma membrane/PVM extensions. RESA export begins simultaneously, within minutes of invasion. In the hours following, the export-associated foci move to evenly surround the parasite, first as smaller clusters that often adopt a ‘ring-like’ structure and then as discrete foci, through which PEXEL-dependent protein export will ultimately travel. Figure 7: Model of export from the ring-stage malaria parasite. Immediately following invasion, dense granule fusion causes local membrane extension and deposits export-associated regions as clusters of foci at the parasite periphery. Each focus contains multiple PTEX complexes as well as non-biochemically associated proteins, such as EXP1. Labelled regions tend to localize at the connexion point to PVM whorl-like extensions and at the tips of pseudopodia-like plasma membrane/PVM extensions. RESA export begins simultaneously, within minutes of invasion. In the hours following, the export-associated foci move to evenly surround the parasite, first as smaller clusters that often adopt a ‘ring-like’ structure and then as discrete foci, through which PEXEL-dependent protein export will ultimately travel. Full size image Following erythrocyte invasion the dynamic nature of ring stages [30] depends on the breakdown of key structural features, including microtubules attached to the inner membrane complex (IMC). IMC degradation is rapid, occurring within 10 min of invasion. Indeed, cupping and flattening of the parasite following invasion to the discoid and amoeboid-like forms seen in previous studies [29] , [30] , [34] occurs during this period. Simultaneously, dense granule fusion with the periphery deposits the organelle contents at, and causes localized whorl-like extensions within, the PVM [29] , [35] . Whether these extensions have some biological role is unclear; however, our data show they exist in parasites of all stages of morphological transition. EXP2 sits between the main parasite body and these membrane extensions, in areas from which the PV marker RAP1 is excluded raising interest for future studies in the possible membrane fusion events occurring at such sites. Core PTEX components EXP2 and HSP101 arrive at the periphery within minutes of invasion, the timeframe on which export begins. HSP101 showed predominant localization to EXP2-defined regions of the PVM but also labelled broadly through the parasite consistently through the lifecycle. This localization may reflect continuous HSP101 translation and trafficking or may signal the role of HSP101 in cellular processes distinct from its involvement in the PTEX complex. Another PTEX component, TRX2, has also been shown to have dual localization to the PVM and another organelle [36] . EXP2 initially labelled large clusters that localized, often asymmetrically, around the parasite periphery. Clusters first spread more evenly around the parasite, then dispersed as individual foci. This finding may suggest that fusion of multiple dense granules occurs at particular sites in the membrane or that many EXP2-labelled foci originate from a single dense granule. The broadly predicted diameter of these EXP2 foci was in the order of 200 nm. The known size of translocation machineries in other systems is surprisingly consistent, despite variation in design and function. Electron microscopy analysis of core components of TOM and the translocase of the outer chloroplast membrane (TOC) complexes suggest outer pore complex diameters of ~16 and 12–14 nm, respectively [37] , [38] . Similarly, HlyE, to which EXP2 shows structural similarity by modelling [16] , forms pores with an outer diameter of 7–12.5 nm [39] , [40] , [41] . HlyE is suggested to form a 13-mer pore from its 34 kDa monomers, with a total homo-oligomeric mass of ~475 kDa [39] . Comparatively, blue native-polyacrylamide gel electrophoresis analysis of EXP2 suggests homo-oligomeric species of ~600 and ~700 kDa [17] . Despite the larger mass of EXP2 oligomers, this suggests a pore with outer diameter of <20 nm, 10fold smaller than our crude estimates of foci size. Therefore, each focus of EXP2 labelling most likely contains numerous PTEX complexes, a conclusion consistent with recent analysis of mitochondrial TOM complexes [24] . This fits with a model by which PEXEL containing exported proteins are trafficked directly to specific zones within the PV containing multiple functional PTEX complexes, thus allowing efficient export [42] . Of note, the TOM complex demonstrates dynamics in clustering upon change of physiological conditions [24] . Individual EXP2 foci remained a relatively constant size using our measurement conditions, suggesting that EXP2 clustering dynamics are modulated at a higher level by movement of entire foci. Despite no previous indication of direct interaction, our findings show a close proximity between EXP1 and EXP2 at the PVM during ring stages, although the segregation of EXP1 becomes less distinct in later time points. Interestingly, both proteins were found in the same DRM sucrose fraction in ring-stage parasites but in separate fractions during schizont stages, possibly reflecting this altered localization [16] , [32] . RAP1, however, also present in the same ring-stage sucrose fraction among others, often appeared to be excluded from EXP2-labelled regions and, at the least, showed a very different labelling distribution. Given the model our data supports, identification of proteins localizing to PTEX-marked PVM domains could signal a possible role in export. In this way, EXP1 appears as a protein of interest for further biochemical investigation. The findings also illuminate a key advantage for high resolution imaging as a tool for identification of molecules that warrant further study. Ultimately, to be considered a translocon, evidence that the PTEX complex interacts with exported proteins at their point of export is essential. The nature of protein export systems makes imaging analysis by immunofluorescence a difficult task under native conditions. Indeed, imaging of cargo proteins has relied almost invariably on mutant versions precluding complete translocation or otherwise perturbed systems. Similar to other systems, export from P. falciparum involves unfolding of cargo proteins and the presence of molecular chaperones [15] , thus altering and masking antibody epitopes. Transit in other systems is rapid, with estimates of chloroplast import of up to 40 000 molecules per chloroplast per minute and translocation occurring at approximately the speed of translation [43] , [44] . Although further details on export kinetics in P. falciparum are lacking, it stands to reason that build-up of cargo protein in native conditions is unlikely. Consistent with this, when fixed from native conditions, association between EXP2 and proteins undergoing PEXEL-dependent trafficking, specifically PfEMP3 and a GBP130 fusion protein, remained ultimately inconclusive, despite localized regions of association between putative cargo and putative translocon. Conversely, imaging of RESA, which localizes to dense granules before invasion and therefore forms a natural concentration upon export [35] , and a reporter protein perturbed from export via a DHFR tag (GBP130-DHFR-GFP) both showed clear association, although not usually direct overlap, with EXP2-labelled PVM regions. Of note, labelling of cargo protein in both conditions associated directly with the intra or extra parasitic faces of EXP2 foci, as distinct from regions of adjacent PV/PVM, adding weight to the idea that we are visualizing functionally relevant exporting protein. In cases where RESA labelling was seen to straddle both sides of a single EXP2 fluorescent foci, a region existed central to the EXP2-labelled foci in which no cargo labelling was seen, suggesting that, at least within the microenvironment of the translocon, recognition of cargo by antibodies is not possible. Therefore, it is likely that we are identifying regions of folded protein build-up occurring upon entry to, and exit from, sites of export. Supporting this, protein unfolding provides the rate-limiting step for import into mitochondria [45] . In the case of GBP130-DHFR-GFP protein that has been perturbed from unfolding, inhibited cargo may ultimately undergo a form of shunting from the translocon either into the PV or PVM, explaining inhibited protein distribution around the parasite in later time points, the lack of inhibited protein export upon removal of WR and unperturbed native protein export after addition of drug [15] . Together, our data strongly support the presence of PTEX in distinct regions of the PV/PVM associated with protein export. Disruption of this trafficking pathway, or indeed the structured PVM domains through which the trafficking occurs, may provide an effective method for simultaneous functional disruption of hundreds of virulence factors. Ethics statement The culture of P. falciparum parasites using donated blood and serum from the Australian Red Cross Society has been approved by The Walter and Eliza Hall Institute Human Ethics Committee (HEC 86/17). Parasite culture and sample preparation Various P. falciparum lines derived from 3D7 and D10 were maintained as asexual stages in erythrocytes (Blood Group O) under standard culture conditions: D10-PfM3′ (ref. 46, ), 3D7+PTEX-150HA and 3D7+HSP101HA for imaging of PTEX [16] , 3D7+GBP130-mDHFR-GFP for export inhibition experiments [15] . To ensure synchronization of parasites, viable filtered merozoites were prepared as described previously [25] . Briefly, late schizont parasites (>40 h), synchronized using either sorbitol or heparin [25] , were purified by magnet (MACS Miltenyi Biotech) and returned to culture in the presence of 10 μ M E-64 protease inhibitor (Sigma). After incubation for 6–8 h, E-64-treated schizonts were pelleted at 1,900 g for 5 min. Parasites were resuspended in culture medium without Albumax II for time points <30 min, but using complete medium with Albumax II (Life Technologies) for >30 min. Following filtration through a 32 mm, 1.2 μm syringe filter (Sartorius Stedim Biotech) merozoites were mixed with washed erythrocytes and allowed to invade, with shaking, at 37 °C. Between 30 and 60 min post invasion (for time points >30–60 min) newly infected cultures were resuspended in fresh culture media and returned to standard culture conditions. Immunofluorescence assays Sample fixation and IFA were undertaken in solution as described previously [31] , [47] . Fixation was in 4% paraformaldehyde with 0.0075% glutaraldehyde in PBS for 30 min at room temperature. Following 10 min permeabilisation using 0.1% Triton-X 100, samples were blocked in 3% bovine serum albumin in PBS at 4 °C overnight. Primary antibodies were used at the following dilutions in blocking solution for 1 h: rabbit anti-EXP2 1:100–1:500 ( [17] ), mouse anti-EXP2 1:500 (ref. 48 ), mouse anti-RAP1 1:500 (ref. 27 ), rabbit anti-MSP1-19 1:200 (ref. 26 ), mouse anti-RON4 1:500 (ref. 49 ), rabbit anti-RON4 (ref. 50 ), mouse anti-RESA 1:100 (ref. 35 ), mouse anti-GFP 1:200 (Roche) and rat anti-HA 1:100 (Roche, Clone 3F10). Following three washes of PBS, AlexaFluor 488 or 594 goat anti-rabbit, rat or mouse (Invitrogen) secondary antibodies were diluted at 1:500 in blocking solution. Following three further washes with PBS, samples were settled onto polyethyleneimine-coated coverslips and mounted in VectaShield (Vector Laboratories) with 0.1 ng μl −1 4′,6–diamidino-2-phenylindole (Invitrogen). Widefield deconvolution and three-dimensional structured illumination (3D-SIM) microscopy For widefield and 3D-SIM microscopy, samples were prepared by IFA as above. Widefield images were captured with mercury illumination on an AxioVert 200M inverted microscope (Zeiss), equipped with a Plan-Apochromat 100 × /1.40 NA Ph3 oil-immersion objective lens (Zeiss), high-efficiency filter sets (Zeiss; in nm: Ex 365-Em 445/50, Ex 470/40-Em 525/50 and Ex 587/25-Em 647/70) and a 1,388 × 1,040 pixel AxioCam Mrm camera (Zeiss) driven by Axiovision release 4.8.2 software (Zeiss). Z-stacks were taken well above and below parasites using a 200 nm Z-step size. Deconvolution (fast iterative setting) and channel shift correction, as measured using commercially available test slides, were performed with an offline 64-bit version of Axiovision release 4.8.1.0 software (Zeiss). 3D-SIM images were captured on a V3 DeltaVision OMX 3D-SIM imaging system (OMX V3) or a DeltaVision OMX 3D-SIM imaging system with a Blaze SIM module (OMX Blaze) (Applied Precision Inc). Solid-state lasers (405, 488, 593 nm) provided wide-field illumination and multi-channel images were captured simultaneously using three cameras (OMX V3, Photometrics Cascade (Photometrics) back-illuminated EMCCD cameras (>90% QE) with a 512 × 512 pixel CCD (charge-coupled device), and on-chip charge multiplication; OMX Blaze, pco.edge scientific CMOS cameras (PCO AG), 512 × 512 pixel with 15-bit dynamic range). Data was captured using either a 100 × (OMX V3) or 60 × (OMX Blaze) 1.4 NA UPlanSApo oil objective (Olympus Corp) and standard excitation and emission filter sets (in nm, 405 EX/ 419–465 EM, 488 EX/500–550 EM and 592.5 EX/608–648 EM). Interference patterns for 3D-SIM were generated either by a physical grid in OMX V3 (refs 51 , 52 ) or by interfering light beams in OMX Blaze [53] . 3D-SIM images were sectioned using a 125 nm Z-step size. Raw 3-phase images were reconstructed as previously described [51] , [52] . General Image Processing Reconstructed 3D-SIM images were rendered in 3D, with interpolation, using IMARIS version 7.2.2–7.6.0 (Bitplane Scientific), with correction for channel-dependent pixel shifts. Full imaging data sets are available on request. For clarity of display, gamma settings were altered on some 3D data sets; however, no comparisons of labelling levels were made from such altered images. General image handling was undertaken using ImageJ ( http://rsb.info.nih.gov/ij/ ) and Photoshop CS5 (Adobe) software before being compiled using Illustrator CS5 (Adobe). Image Analysis Analyses were undertaken on 3D-SIM data sets in 3D using IMARIS versions 7.2.2–7.6.0 (Bitplane Scientific). Statistical presentation and analyses were performed using Prism version 5.0a (Graph Pad Software). For colocalization studies, IMARIS ‘Colocalization Module’ was used. To avoid subjectivity all thresholds were automatically determined using algorithms based on those of Costes [54] . To create a stringent threshold, the automated algorithm was run only on values above an initial input pixel intensity value of 1,000 in the non-EXP2 channel, determined after consideration of representative images from each data set. The % colocalization (‘Intensity Weighted Overlap’ statistic) was calculated as the percentage of summed pixel intensities in the non-EXP2 channel that coincide with above threshold EXP2 values. A Kruskal–Wallis test, with Dunn's multiple comparison post test, was used to analyse the difference of medians between all data sets depicted in Fig. 2d . As required, all data sets showed similar variance by Levene’s test [55] . As a precaution, a non-parametric test was used because some samples did not pass the D’Agostino and Pearson omnibus normality test. Similar analysis was performed for data presented in Fig. 4c ; however, GBP130-DHFR-GFP data was excluded from analysis due to its non-similar distribution, again measured using Levene’s test. EXP2 volume analyses were performed using parasites labelled for RAP1 and EXP2. Using IMARIS ‘Surface tool’, ‘Pre-segmentation’ EXP2-labelled regions were isolated using automated thresholding based on a published algorithm [56] (0.0395 μm smoothing, Background subtraction 0.29625 μm, automatic threshold). Objects with <20 voxels were discarded as they were smaller than the minimum resolvable volume of the microscope. Regions of EXP2 entirely outside the RAP1-labelled region (0.395 μm smoothing, absolute intensity, automatic thresholding) were also discarding to prevent inclusion of non-specific EXP2 fluorescence. Following masking of the original EXP2 data with the ‘Pre-segmentation’ EXP2 surface, this data was re-analysed by applying a new threshold for ‘Segmented’ regions (no smoothing, absolute intensity, automatic thresholding). This time objects were split using a region-growing algorithm, with central ‘seed points’ identified using an estimated diameter of 0.118 μm, based on the maximum resolution of the microscope and deemed reasonable through testing of representative data. Again, objects <20 voxels were discarded. Volume of objects was used as a measure of labelled region size. Electron Microscopy Infected erythrocytes were prepared as described above and fixed with 2.5% glutaraldehyde in 0.1 M sodium cacodylate, rinsed and postfixed in reduced Osmium tetroxide, en bloc stained with aqueous uranyl acetate and Walton’s lead aspartate and embedded in LRWhite. Sections (200 nm) were cut and observed in a Tecnai F30 (FEI, Heindoven, The Netherlands). Micrographs from serial sections were aligned by cross correlation and corrected for directional shift. Regions of interest were segmented by manual tracing [57] using the IMOD package [58] , [59] . How to cite this article: Riglar D.T. et al . Spatial association with PTEX complexes defines regions for effector export into Plasmodium falciparum -infected erythrocytes. Nat. Commun. 4:1415 doi: 10.1038/ncomms2449 (2013).